A hybrid CMOS-imager with a solution-processable polymer as photoactive layer The solution-processability of organic photodetectors allows a straightforward combination with other materials, including inorganic ones, without increasing cost and process complexity significantly compared with conventional crystalline semiconductors. Although the optoelectronic performance of these organic devices does not outmatch their inorganic counterparts, there are certain applications exploiting the benefit of the solution-processability. Here we demonstrate that the small pixel fill factor of present complementary metal oxide semiconductor-imagers, decreasing the light sensitivity, can be increased up to 100% by replacing silicon photodiodes with an organic photoactive layer deposited with a simple low-cost spray-coating process. By performing a full optoelectronic characterization on this first solution-processable hybrid complementary metal oxide semiconductor-imager, including the first reported observation of different noise types in organic photodiodes, we demonstrate the suitability of this novel device for imaging. Furthermore, by integrating monolithically different organic materials to the chip, we show the cost-effective portability of the hybrid concept to different wavelength regions. Solution-processable organic photodetectors (OPDs) can be deposited with simple and low-cost process techniques like spin- and spray-coating [1] , which do not involve high temperatures and vacuum. In addition, the liquid state of the semiconductor allows a straightforward deposition on any kind of substrate, including flexible ones [2] , [3] , [4] , [5] and amorphous silicon thin-film transistor circuitry [6] , [7] , as well as combination with inorganic materials, for example colloidal quantum dots as infrared absorbers [8] . In addition, various organic materials absorbing at different wavelengths can be integrated in the photodetector. For the visible range of the spectrum, a bulk-heterojunction of PCBM:P3HT (poly(3-hexylthiophene): [6,6]-phenyl C61 butyric acid methylester) [9] , [10] (refs 9 , 10 ) can be employed for photodetection [11] or squaraine (SQ) [12] for a near-infrared (NIR)-enhanced absorption. High performance and low-cost polymer photodetectors can also be realized beyond the absorption edge of silicon at 1.1 μm competing with resource-limited and costly InGaAs photodiodes [13] . Solution-processability is also the key to develop low-cost hybrid imaging technologies that combine certain advantages of organic materials with technically mature silicon technologies. In previous attempts, organic materials were integrated on active-matrix backplanes with a -Si:H thin-film transistors [6] , [7] , [8] , creating hybrid organic devices like flexible image sensor arrays [7] . Owing to the large pixel size of a -Si:H-devices, which typically exceeds 100 μm ( [6] , [7] , [8] ), they are commercially employed only in large-area applications like X-ray image sensors and (organic) displays, as active-matrix organic light-emitting diodes [14] . For sensing in the visible and NIR range of the spectrum, only two competitive silicon imager technologies for high-pixel resolution are available: complementary metal oxide semiconductors (CMOS) and charge-coupled devices (CCD). Compared with a -Si:H-devices with low-electron mobility μ ( a -Si: μ ~1 cm 2 V −1 s −1 ) [15] , CMOS-imagers ( c -Si: μ ~1,000 cm 2 V −1 s −1 ) provide higher transistor switching speed, which is deployed in high-speed CMOS-imagers with frame rates up to the megahertz range [16] . Additionally, the electronic read-out noise is about a factor of 10 lower for CMOS-sensors (typically 100 electrons or less) compared with a -Si:H-imaging devices [17] . The rivaling CMOS and CCD technology, with different strengths in terms of sensitivity, noise, speed and cost, have to satisfy the need of the market, requiring an increasing number of photoactive pixels on the same chip area. By reducing pixel dimensions, approaching a minimum pixel size of about 1 μm ( [18] ), the light sensitivity of the active pixel sensor (APS), the most competitive CMOS-imager design compared with CCD, decreases. This is due to the incorporation of the read-out amplifier directly into each pixel, which reduces the pixel area available for photon detection. The fraction of this photoactive area compared with the overall pixel size, the so called ‘pixel fill factor’, is usually in the range of only 30% ( [19] , [20] ), which reduces the external quantum efficiency (EQE) by the same amount. To overcome this limit, focusing microlens-arrays are implemented [21] , [22] , the sensor is transformed into a back-illuminated imager [23] , a multilayer of amorphous silicon (‘thin film on ASIC’) [24] , [25] , [26] or thin organic photoconducting materials can be vacuum-deposited [27] . All these methods require significant additional processing and, therefore, increasing cost. We demonstrate here that an organic photoactive layer, deposited by low-cost spray-coating, can replace the silicon and can cover the CMOS-pixel array as a continuous film without a demand for further structuring, creating a hybrid CMOS-imager. As the organic material is vertically integrated and covers the read-out electronics, the pixel fill factor increases up to 100%, and hence also the EQE, which can be as high as about 75% for sprayed OPDs [1] . We realize the fabrication of the first hybrid CMOS-imager consisting of a CMOS-chip fabricated in standard technology and an organic bulk-heterojunction as photoactive layer deposited with a simple spray-coating process. By fully covering the hybrid pixels, featuring a minimum size of 15 μm, which is the smallest size reported so far for a solution-processed photodiode, a 100% pixel fill factor and an EQE up to 50% is reached. To demonstrate the capabilities and suitability of the hybrid technology, a set of optoelectronic measurements are performed, showing for example, high dynamic range (DR; 60 dB), a sufficient frame rate for imaging (bandwidth~15 kHz) and small pixel-to-pixel cross-talk. Furthermore, portability to different wavelength windows is proven by spray-deposition of organic active layers with different absorption spectra. Hybrid CMOS-imager build-up The inorganic part of the hybrid imager, the CMOS-chip, was fabricated in a commercial 0.35 μm CMOS-technology and designed to the needs of the optoelectronic characterization (for a more detailed description see ref. 28 ). To investigate the noise performance of the OPD, a low-noise charge amplifier was implemented in the read-out electronics. Considering the area needed for this amplifier and to avoid read-out channel non-uniformities, a passive pixel configuration [20] was chosen. For the read-out with the charge amplifier, the pixel has to be selected by a row decoder and column multiplexer. With the addition of a second charge amplifier to the read-out electronics, two pixels can be addressed at the same time, enabling pixel-to-pixel cross-talk measurements. The pixels with different pad sizes ranging from 50 μm down to 15 μm are arranged in different arrays, the largest one with 30 × 30 pixels is also suitable for acquiring low-resolution images, see Fig. 1a . In the hybrid approach, in contrast to a standard CMOS-imager, the whole pixel is covered with a metallization layer so that the full pixel area can be employed for the OPD. The fully CMOS-compatible aluminum layer, used here, has to connect the read-out electronics to the organic photoactive layer, therefore, acting also as the bottom electrode of the OPD. 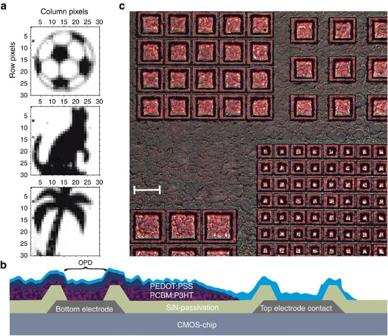Figure 1: Device structure and low-resolution images. (a) The monochrome images, showing a football, a cat and a palm, are acquired by the 30 × 30 pixel array (top-view showed inFig. 1cwith 15 μm sized pixels under ambient light). Dark and gain corrections were performed as described in the Methods. (b) The side view of the layer structure starts with the CMOS-chip, an electrically insulating silicon nitride (SiN) layer and the aluminum layer as bottom electrode for the OPDs, followed by the photoactive PCBM:P3HT blend, a hole-conducting layer (darker blue) and a highly conductive anode (lighter blue) consisting both of PEDOT:PSS as described in the Methods. The indicated rough structure of the organic layers arises because of the spray-deposition method. (c) The top-view of the hybrid imager, showing the different arrays with pixels of different sizes and pitches. The length of the scale bar in the picture is 50 μm. The pixel size in the upper part is 35 μm, at the bottom 50 μm, the larger array consists of 15 μm big pixels used to acquire the low-resolution images inFig. 1a. The pink-coloured sprayed organic layer that covers the pixels is the PCBM:P3HT bulk-heterojunction. Figure 1: Device structure and low-resolution images. ( a ) The monochrome images, showing a football, a cat and a palm, are acquired by the 30 × 30 pixel array (top-view showed in Fig. 1c with 15 μm sized pixels under ambient light). Dark and gain corrections were performed as described in the Methods. ( b ) The side view of the layer structure starts with the CMOS-chip, an electrically insulating silicon nitride (SiN) layer and the aluminum layer as bottom electrode for the OPDs, followed by the photoactive PCBM:P3HT blend, a hole-conducting layer (darker blue) and a highly conductive anode (lighter blue) consisting both of PEDOT:PSS as described in the Methods. The indicated rough structure of the organic layers arises because of the spray-deposition method. ( c ) The top-view of the hybrid imager, showing the different arrays with pixels of different sizes and pitches. The length of the scale bar in the picture is 50 μm. The pixel size in the upper part is 35 μm, at the bottom 50 μm, the larger array consists of 15 μm big pixels used to acquire the low-resolution images in Fig. 1a . The pink-coloured sprayed organic layer that covers the pixels is the PCBM:P3HT bulk-heterojunction. Full size image As photoactive layer, a bulk-heterojunction of P3HT:PCBM (poly(3-hexylthiophene): [6,6]-phenyl C61 butyric acid methylester), absorbing in the visible range of the spectrum, was chosen. Alternatively, also SQ was added for NIR-enhanced absorption. To decrease the dark current, a layer of PEDOT:PSS (poly(3,4-ethylenedioxythiophene):poly(styrenesulfonate)) was included to the organic stack on the chip. As this organic material combination is usually inserted in a bottom absorbing photodetector [11] , with a low work function metallization like aluminum as top electrode, an inverted OPD fabrication process had to be developed to generate a top-absorbing detector [29] , [30] suitable for integration on the CMOS-chip. As highly transparent top anode, a conductive formulation of PEDOT:PSS was deposited as uppermost layer [30] . In Fig. 1b a simple sketch of the layer structure of the hybrid imager is shown. All organic layers are solution-processable and were deposited with an automatic air atomizing spray gun (see Methods). This vertical deposition method was chosen because of the small chip size (2 × 2 mm 2 ) and the high texture of the CMOS-chip, which can hamper a homogenous material deposition performed with lateral methods like spin-coating or doctor-blading. Spraying parameters were optimized to obtain small drop sizes (5–10 μm), see Fig. 1c , and, therefore, small layer roughness (root-mean-square value~100 nm) to minimize non-uniformities of the organic layer thickness. Dark and illuminated current-voltage characteristics As a charge amplifier with a feedback capacitance C is chosen for the signal read-out, the corresponding output is a voltage V proportional to the amount of charge Q integrated over a certain integration time t int, V= Δ Q(t int )/C , which can be transformed to a current I by using Δ Q(t int )=I Δ t int . 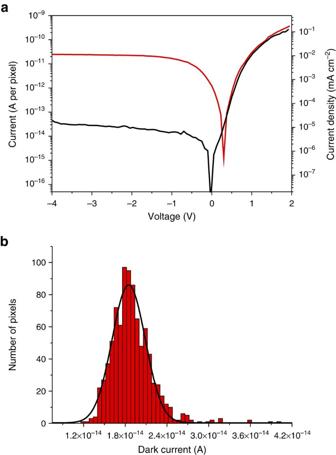Figure 2: The voltage-current characteristic of the hybrid imager. (a) The current versus the voltage characteristics of a single pixel with 15 μm pad size. The curves refer to bothyaxes, showing the absolute current per pixel, as well as the respective current density. The upper (red) curve represents the photocurrent, measured under illumination of 70 μW cm−2at a wavelength of 535 nm. Below, the photodiode dark current is shown (black). (b) The distribution of the dark currents of all pixels (pad size 15 μm) in a 30 × 30 pixel array measured at an external bias of −1.5 V. The data is fitted assuming a Gaussian distribution. Figure 2a shows a typical IV -curve of a pixel of the hybrid imager with 15 μm pad size under dark and illuminated conditions. At a power density of 70 μW cm − 2 of monochromatic light at 535 nm, the current increases by about three orders of magnitude. The rectification ratio of the dark current at bias voltages of ±2 V is 12,000. This value is twice as high as reported by Rauch et al . [8] for a hybrid organic diode on an a -Si:H matrix backplane. The superior low dark current, to our knowledge the best ever reported for a sprayed organic photodiode, ranges from about 15 fA per pixel (7 × 10 −6 mA cm − 2 ) at −1.5 V to about 50 fA per pixel (2 × 10 −5 mA cm − 2 ) at −4 V. This result is within the full width at half maximum (FWHM) of the Gaussian distribution of all pixels with 15 μm pad size contained in the 30 × 30 array, showed in Fig. 2b for an applied voltage of −1.5 V. The average dark current of all these pixels is about 20 fA, with a FWHM of about 6 fA. This dark current distribution appears as so called fixed-pattern noise (FPN) in the output signal of the hybrid imager and is generated by OPD non-uniformities, like layer thickness variations. We can exclude chip non-uniformities as a passive pixel configuration, with a shared read-out electronic for all pixels, is used. Despite the thickness variations of the sprayed organic layers, the resulting dark FPN, which is usually expressed as voltage variation for a typical integration time at video rate, resulting in FPN=1.2 mV for FWHM( I )=6 fA and t int =20 ms (with V= ( I t int ) /C and amplifier capacitance C= 100 fF), is quite low as it is comparable with the fundamental temporal noise, which is addressed in the following section. Figure 2: The voltage-current characteristic of the hybrid imager. ( a ) The current versus the voltage characteristics of a single pixel with 15 μm pad size. The curves refer to both y axes, showing the absolute current per pixel, as well as the respective current density. The upper (red) curve represents the photocurrent, measured under illumination of 70 μW cm − 2 at a wavelength of 535 nm. Below, the photodiode dark current is shown (black). ( b ) The distribution of the dark currents of all pixels (pad size 15 μm) in a 30 × 30 pixel array measured at an external bias of −1.5 V. The data is fitted assuming a Gaussian distribution. Full size image Noise properties and DR The operational range of the hybrid imager is described by the DR that quantifies the ability of the sensor to adequately image both high light intensities and dark shadows in a scene. DR is defined as the ratio between the maximum and minimum detectable signal, DR=20log( V max / V min ). With the hybrid imager, the maximum voltage signal due to light illumination that can be read-out is about 2 V, which is limited by the amplifier operational range. The minimum signal is related to the residual noise under dark conditions. The photodiode dark current generates two types of noise, the already discussed FPN, which can be corrected by image post-processing (as in Fig. 1a ) and the temporal noise, which refers to time-dependent signal fluctuations setting a fundamental limit on image sensor performance. Apart from thermal noise sources due to pixel electronics (for example, amplifier noise and pixel reset noise) for a CMOS-sensor the dominant dark noise type is shot noise. It is the root-mean-square value of the dark voltage signal following a Poisson distribution, with the number of leakage carriers N , due to the discrete and independent motion of carriers and is given by: with e the elementary charge and C the charge amplifier feedback capacitance. With C =100 fF and depending on the integration time, shot noise voltages below 2 mV (for signal voltages V <2 V) are expected. For organic photodiodes, Gong et al . [13] assumed shot noise as major contribution although no investigations about different noise types are reported so far to our knowledge. In contradiction to this expectation, the hybrid imager dark noise measurements (for details see Methods) reveal results deviating from shot noise behavior. In Fig. 3a the RMS-noise voltage deviation of a hybrid pixel for different output dark currents (obtained by applying different external bias voltages) and integration times is shown. 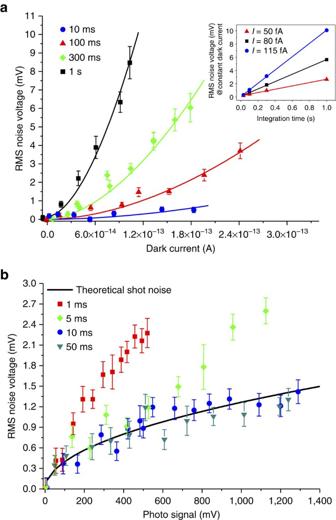Figure 3: Measurement of the dark and photon root-mean-square-noise voltages for different charge integration times. (a) The dark current s.d., expressed as noise voltage, versus the dark current, which was varied by applying different external voltages. The error bars represent the s.d. of a set of noise voltage measurements. The fitting was done assuming an approximate quadratic dependence on the dark current. The inset shows the linear increase of the noise voltage with different integration times and constant dark currentI. (b) The change of the photocurrent and the corresponding photon noise voltage signal was achieved by varying the light power of a green light-emitting diode (535 nm). The external applied bias was kept constant at −1.5 V. The corresponding dark signal was subtracted from the data. While for t int =10 ms the noise level stay well below 1 mV, increasing the dark current lead to a noise level increase of about one order of magnitude for t int =1 s. The strong impact of integration time hints to a dominant flicker noise contribution, which is proportional to the current I and frequency f ( [31] ): Figure 3: Measurement of the dark and photon root-mean-square-noise voltages for different charge integration times. ( a ) The dark current s.d., expressed as noise voltage, versus the dark current, which was varied by applying different external voltages. The error bars represent the s.d. of a set of noise voltage measurements. The fitting was done assuming an approximate quadratic dependence on the dark current. The inset shows the linear increase of the noise voltage with different integration times and constant dark current I . ( b ) The change of the photocurrent and the corresponding photon noise voltage signal was achieved by varying the light power of a green light-emitting diode (535 nm). The external applied bias was kept constant at −1.5 V. The corresponding dark signal was subtracted from the data. Full size image Flicker noise is known to be present in many electronic devices, as the origin is related to a slow fluctuation of properties of the materials used in the device. For organic photodiodes, little is known about flicker noise, differently from inorganic metal-oxide-semiconductor field-effect transistors (MOSFETs) [32] and organic thin-film-transistors [31] , [33] , [34] , [35] , where flicker noise is observed for the drain current. Here, the two dominant flicker noise sources described are trapping–detrapping of carriers at the gate oxide (causing a carrier number fluctuation) and bulk scattering (causing a mobility fluctuation). Recent publications hint to various types of traps within the disordered, amorphous organic semiconductor, like at grain-boundaries [34] , [35] , not only at the gate oxide. Similar mechanisms could apply for the organic photodiodes, but for a detailed understanding an in-depth investigation and simulations including the various trap species are necessary. The experiment shows a linear dependence of the noise voltage on the integration time in the inset of Fig. 3a , proving that β =1, which indicates an uniform distribution of trap energies [36] . The dependence on the dark current, fitted quadratically in Fig. 3a , indicates that α →2, hinting to dominant volume trapping instead of a surface nature [37] . Regarding the impact on imaging, the high flicker noise for integration times in the range of 1 s is not detrimental as for most imaging applications integrations times are in the millisecond range. The DR of the hybrid detectors can be henceforth estimated to about 60 dB, assuming 2 mV as minimum detectable dark signal for integration times smaller than 100 ms. As detection of N photons is a random process obeying Poisson statistics, equation (1) accounts for the photon shot noise, as well. It presents the fundamental limit in the signal-to-noise ratio. In Fig. 3b , noise voltage measurements of the hybrid imager performed under varying illumination and with typical integration times for imaging (1 ms to 50 ms) are shown. In contrast to the dark signal, the results are much closer to the theoretical shot noise, also included in the graph, and behave differently: while for integration times ≥10 ms the noise voltage match the photon shot noise, decreasing the integration time increases slightly the noise level. This can be due to an additional noise component associated with the high current flowing in the device due to illumination. Possibly, the origin of this behavior is related to charge accumulation at the blend-PEDOT:PSS interface and a related change of the electric field in the device as observed for similar devices structures before [29] , [30] . The related electric field dependence of the mobility [38] , [39] could account for the flicker noise component as well. External quantum efficiency The EQE of the photocurrent, the ratio between generated electrons and incident photons on the pixel area, will not be reduced by the amount of photo-insensitive electronics inside the pixel of the hybrid imager as the photoactive material is placed on top of it. The spectral dependent EQE of a typical pixel (15 μm pad size) of our hybrid imager for different applied voltages is shown in Fig. 4a . The spectral maximum of >40% for bias voltages larger than −1.5 V can be found around 420 nm, although the EQE stays quite constant in the visible range of the spectrum up to the absorption edge of PCBM:P3HT at around 650 nm and would allow, therefore, the separation of the three primary colors with additional filters. The average EQE ( Fig. 4b ) of all pixels in the 30 × 30 array stays at about 40%, although single pixels exhibit EQEs up to 50%. The thickness of the photoactive layer strongly influences the EQE, as shown in the Supplementary Discussion and Supplementary Fig. S1b , resulting in an EQE decrease of typically 5% with a thickness increase of about 100 nm. As the roughness of the sprayed layer is about 100 nm, large EQE variations are expected. The FWHM of the assumed Gaussian distribution in Fig. 4b a measure of the photoresponse non-uniformities, is about 9% EQE. This value is higher compared with conventional silicon imagers but can be mostly compensated with electronic post-processing [40] . The average photoactive layer thickness (about 650 nm) in the hybrid imager is chosen to be slightly higher than the optimum for maximum EQE to ensure the low uniform dark current in Fig. 2b in spite of layer thickness fluctuations (see Supplementary Fig. S1a for the influence of layer thickness on the dark current). Still, the achieved EQE of the hybrid imager is better than that of most standard front-side illuminated APS imagers, which is usually below 30% ( [19] , [20] ). 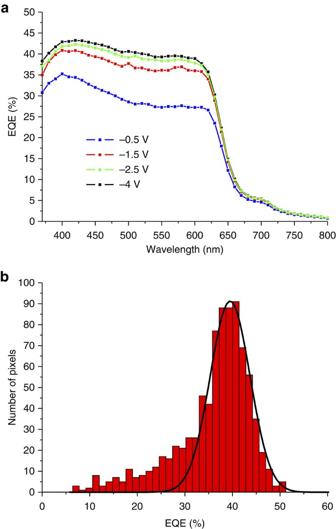Figure 4: EQE of the hybrid imager. (a) A typical spectral EQE for a single pixel with 15 μm pad size is shown for different external applied voltages. (b) The asymmetric distribution of the EQE of all pixels (pad size 15 μm) in a 30 × 30 pixel array, measured at an external bias of −4 V, overlaid by a Gaussian fit. Figure 4: EQE of the hybrid imager. ( a ) A typical spectral EQE for a single pixel with 15 μm pad size is shown for different external applied voltages. ( b ) The asymmetric distribution of the EQE of all pixels (pad size 15 μm) in a 30 × 30 pixel array, measured at an external bias of −4 V, overlaid by a Gaussian fit. Full size image Cross-talk between pixels The downscaling of organic photodiodes to pixel sizes suitable for commercial imaging application (pad sizes ≤10 μm) and the increase of the number of pixels per area requires knowledge about the cross-talk between adjacent pixels as it limits the minimum feasible spacing in between the pixels. Compared with the pixel fill factor, the overall chip fill factor takes this inter-pixel area into account and cannot be increased to 100% due to cross-talk. To quantify the amount of signal collected by neighboring pixels in the hybrid imager, a green light-emitting diode (535 nm) was focused with an objective on a single pixel (pad size 15 μm, pitch 30 μm) and the generated photocurrent as well the signal of a neighboring pixel were read-out simultaneously by the two charge amplifiers. In Fig. 5 the cross-talk between the pixels, at an applied external bias of −3.5 V, is illustrated, distinguishing between close (vertical plus horizontal) and diagonal neighbors. The signal of the outside pixels is on the dark current level. Including all neighboring pixels, the cross-talk is 0.165% of the illuminated pixel signal (close neighbors: 0.258%, diagonal neighbors: 0.072%). By reducing the applied voltage to −1.5 V, the cross-talk is slightly increased to 0.182% (close neighbors: 0.368%, diagonal neighbors: 0.114%). These very low values imply that both electrical cross-talk (related to photocarrier diffusion across the organic layers) and optical cross-talk are well suppressed. Generally, optical cross-talk is expected to be low due to the high absorption coefficient in organic photoactive layers [41] , but a residual contribution could be related to photons guided inside the encapsulation glass sheet and directed towards an adjacent pixel. The electrical cross-talk should be well suppressed by the low mobility of organic bulk-heterojunctions (~1 × 10 −4 cm 2 V −1 s −1 ) [42] . In addition, the high aspect between pixel-to-pixel distance (~25 μm, including the contribution of the additional bulges of the silicon nitride (SiN)-passivation layer) and the photodiode stack thickness (~1 μm) is also favorable for the measured low-cross-talk in our hybrid imager. 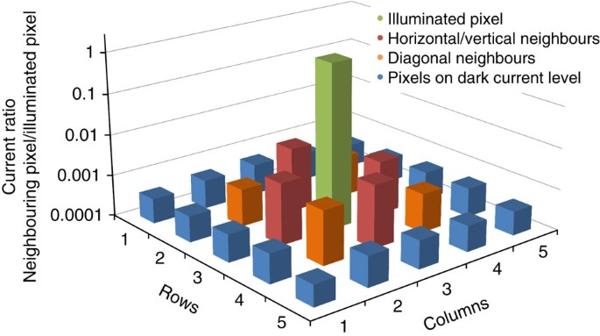Figure 5: Cross-talk between neighboring pixels. The ratio of photocurrent, created in the central illuminated pixel on a semi-logarithmic scale, which reaches adjacent pixels. The pixel pad size is 15 μm, the pitch 30 μm. The applied external bias is −3.5 V and the light power is about 450 μW cm−2(535 nm). Figure 5: Cross-talk between neighboring pixels. The ratio of photocurrent, created in the central illuminated pixel on a semi-logarithmic scale, which reaches adjacent pixels. The pixel pad size is 15 μm, the pitch 30 μm. The applied external bias is −3.5 V and the light power is about 450 μW cm − 2 (535 nm). Full size image Detector speed For conventional imaging application typical frame rates are around 100 frames/s as typical integration times and data transfer times, which are both in the order of milliseconds, limit the speed of the detector. Investigating the speed of the OPDs (with different pad sizes) in the hybrid imager by measuring the response time of the photocurrent due to illumination with pulsed light, shows that typical rise and fall times τ of the signal are in the order of 10–15 μs. These values correspond to a bandwidth 1/(2πτ) of about 10–15 kHz, which is sufficient for imaging. Solution-processed OPDs can actually be even faster [1] , [30] , [43] , making them suitable also for high-speed imaging applications like line scan cameras for industrial imaging (~100 kHz). Acquisition of monochromatic test images To validate the hybrid imager concept, several low-resolution images (30 × 30 pixels), see Fig. 1a , of simple objects were acquired under ambient light conditions, focusing the light with an objective on the pixel array. The large variation of the sensitivity among the pixels was homogenized by performing a dark and a gain correction (see Methods). Only about four pixels in Fig. 1a remain darker than the surrounding bright background because of higher leakage current. Portability to different wavelength ranges The major strength of the hybrid concept is the portability to different solution-processable photoactive materials. To demonstrate the ease of switching the material system to extend the absorption to the NIR region, we added a SQ dye [12] , [44] , [45] , [46] as additional donor material to the PCBM:P3HT solution to exploit the absorption spectrum of SQ between 600 and 900 nm. About solar cells and photodetectors with a bulk-heterojunction active layer of PCBM:SQ, it was already reported [44] , [45] , [46] . In the Supplementary Discussion we report about the fabrication of large scale reference photodetectors to determine an optimal mixing ratio for a PCBM:P3HT:SQ detector. For the hybrid imager, we sprayed the optimized PCBM:P3HT:SQ solution on the chip without any change of process parameters or of the imager build-up. The absorbance spectrum of this panchromatic organic material is shown in Fig. 6a , generated by the three different materials P3HT, PCBM and SQ. The measured dark currents of the chip proved to be similar to the pure PCBM:P3HT hybrid imager, 26 fA per pixel (1.2 × 10 −6 mA cm − 2 ) at −1.5 V. To validate this sensor, simple images were acquired at two different wavelengths as shown in Fig. 6b . At 530 nm, only the PCBM:P3HT is sensitive to the light. At 850 nm, in addition to the SQ, there is also a small contribution of the collection of diffusing photocarriers generated in the silicon substrate. As shown in Supplementary Fig. S3 and the Supplementary Discussion , the influence of the silicon can be neglected, as the pure PCBM:P3HT hybrid imager is almost blind at this wavelength. 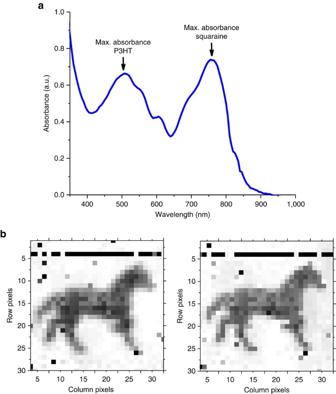Figure 6: Change of the spectral sensitivity of the hybrid detector by adding SQ. (a) The absorbance spectrum of the panchromatic organic photoactive layer with PCBM, P3HT and SQ. (b) Images, showing a horse, taken by the corresponding hybrid CMOS-detector. The left one is acquired by illumination with green light (535 nm), the right one with a NIR-light-emitting diode at 850 nm. Figure 6: Change of the spectral sensitivity of the hybrid detector by adding SQ. ( a ) The absorbance spectrum of the panchromatic organic photoactive layer with PCBM, P3HT and SQ. ( b ) Images, showing a horse, taken by the corresponding hybrid CMOS-detector. The left one is acquired by illumination with green light (535 nm), the right one with a NIR-light-emitting diode at 850 nm. Full size image The above presented results of the electro-optical device characterization demonstrate the suitability of the hybrid detector for imaging applications, as small dark current densities, high detector speed, a low temporal noise level and small pixel sizes are prerequisites. The state-of-the-art performance of the hybrid CMOS-imager could be obtained by organic layer deposition with a cheap, facile and fast spraying method. We showed that a 100% pixel fill factor is feasible due to the vertical integration of all organic layers on top of the CMOS-chip, resulting in higher EQE as of most standard front-side illuminated APS imagers. Regarding the non-photoactive inter-pixel area, the low pixel-to-pixel cross-talk indicates the feasibility of a strong reduction of the pixel pitch to increase the overall chip fill factor. The addition of a SQ dye to the PCBM:P3HT bulk-heterojunction by blending the three organic materials in a single solution results in an extended hybrid CMOS-imager wavelength range towards the NIR region. This easy portability of the hybrid concept to different absorption spectra, which is a benefit arising due to the solution-processability, could also allow future creation of cheap CMOS-NIR-detectors beyond the absorption edge of silicon (1.1 μm). Besides the use of suitable NIR polymers, also a further device hybridization with organic/nanocrystal composites is feasible [8] , [47] . Deposition of the organic layers on the CMOS-chip Directly before the organic deposition, the CMOS-chip was etched shortly in ammonium hydroxide to remove the native oxide on the aluminum layer used as OPD cathode. For the deposition of all organic materials, a commercially available two-substance nozzle spray gun (Krautzberger GmbH, Germany) was used. The photoactive blend of PCBM:P3HT with a mixing ratio of 1:0.75 was dissolved in the aromatic solvents toluene and 1,2-dichlorobenzene, stirred overnight at 60 °C, and large-area sprayed on top of the CMOS. After a plasma activation of the blend layer (for details see ref. 29 ), the PEDOT:PSS formulation Clevios P VP CH 8000 used as electron blocking layer, diluted in deionized water (PEDOT:PSS: H2O=1:2), was deposited and dried for 5 min at 120 °C. The conductive (sheet resistance~70 Ω per square) and transparent (~85% transmission in the visible range of the spectrum) polymer anode, consisting of the PEDOT:PSS formulation Clevios PH 1000 and ethylene glycol as conductivity enhancer, was sprayed as uppermost layer. In a nitrogen-filled glove box, the last annealing step was performed (140 °C, 10 min), completed by an encapsulation with a glass sheet and epoxy resin to hinder oxygen and water to react with the organic layers. Hybrid imager signal read out A test board was fabricated in order to provide the required power supply and analog reference signals to the CMOS-chip. A microcontroller (NXP LPC1768), also hosted on the test board, was used to generate the required digital timing signals, to perform Analog-to-Digital conversion of the sensor output signal and to handle the data transfer to a PC through a USB interface. Pixel signal acquisition was performed by sampling and digitizing the charge amplifier output at two different time instants: immediately after amplifier reset and at the end of the integration time. The output voltage, proportional to the integrated current, was computed as the difference between the two voltage samples (correlated double sampling), and the current was calculated from the output voltage using integration time and capacitance after proper calibration. In current measurements, each voltage measurement was repeated with different integration times varying from 100 to 100 ms, to account for the current range spanning more than 6 decades. As noise carriers generated inside the substrate can be collected by the transistor junctions acting as switches for connecting the organic photodiode to the amplifier, we employed a correction for the dark current to eliminate this leakage signal. A typical value of the leakage current, regarding an equal amount of switches (number of switches per column varies on the chip), is about 10 fA±2 fA (s.d.). Hybrid imager characterization Photocurrent and single point EQE measurements were performed under illumination with a green light-emitting diode with a wavelength of 535 nm and a power density of 70 μW cm − 2 . The green light-emitting diode was also used for dynamic, photon shot noise and cross-talk measurements. Spectrally resolved EQE measurements were carried out on a dedicated electro-optical setup composed by a white-light source (Oriel model 66183, 200W), a monochromator (Jobin Yvon HR250), a motorized positioning stage and a calibrated silicon detector. Noise measurements were carried out acquiring the chip output signal directly with an oscilloscope (LeCroy wavepro 7200) and performing signal filtering and correlated double sampling operations on the digitized output signal. Total output noise was measured as the s.d. of the sampled output value over a large number (>100) of acquisitions. The noise contributions due to the charge amplifier and the silicon leakage were measured with the photodiodes biased at their open circuit voltage and were subtracted in quadrature from the total measured noise. For dynamic measurements the OPDs were illuminated with square-waved light pulses (about 4 mW cm − 2 , duty cycle 1%) and the corresponding photoresponse was extracted from the time-domain charge integration signal with the oscilloscope by calculating the derivative. To reduce the noise due to the differentiation, the integrated output signal was averaged over a large number of acquisitions (>100) and a low-pass filter with a time constant of 100 ns was applied. As the OPD rise and fall time had a much larger time constant, this operation caused a negligible distortion in the measured pulse response. Imaging The monochromatic images were acquired with the 30 × 30 matrix of hybrid pixels and an objective (focal length: 6 mm, focal ratio: 1.2). The integration time was set to 5 ms. The final images were corrected by subtracting the dark level and by multiplying with the gain factor to compensate the sensitivity in homogeneities among the pixels. The gain factor was defined by the ratio of each pixel raw data signal divided by the corresponding signal obtained by sensing a white sheet of paper under ambient light. How to cite this article: Baierl D. et al . A hybrid CMOS-imager with a solution-processable polymer as photoactive layer. Nat. Commun. 3:1175 doi: 10.1038/ncomms2180 (2012).